Expression and functions of long noncoding RNAs during human T helper cell differentiation Long noncoding RNAs (lncRNAs) regulate an array of biological processes in cells and organ systems. Less is known about their expression and function in lymphocyte lineages. Here we have identified >2000 lncRNAs expressed in human T-cell cultures and those that display a TH lineage-specific pattern of expression and are intragenic or adjacent to TH lineage-specific genes encoding proteins with immunologic functions. One lncRNA cluster selectively expressed by the effector TH2 lineage consists of four alternatively spliced transcripts that regulate the expression of TH2 cytokines, IL-4, IL-5 and IL-13. Genes encoding this lncRNA cluster in humans overlap the RAD50 gene and thus are contiguous with the previously described TH2 locus control region (LCR) in the mouse. Given its genomic synteny with the TH2-LCR, we refer to this lncRNA cluster as TH2-LCR lncRNA. It is estimated that mammalian genomes encode>10,000 unique long noncoding RNAs (lncRNAs) [1] , [2] , [3] , [4] . These RNAs are defined as>200 base pairs in length but have little translation potential due to the presence of numerous stop codons in the mature transcript [5] , [6] , [7] , [8] . Genes encoding lncRNAs are oftentimes defined by their relationships with neighbouring protein-coding genes. Antisense lncRNAs are transcribed in opposite directions from neighbouring coding genes but exhibit some overlap with protein-coding genes such as partial sharing of coding exons. Intronic lncRNAs initiate within the introns of protein-coding genes, do not overlap with protein-coding exons and are transcribed in either orientation relative to adjacent protein-coding genes. Divergent lncRNAs are transcribed in opposite directions relative to promoters of protein-coding genes and usually initiate transcription within a few hundred base pairs of transcriptional start sites of neighbouring protein-coding genes. Intergenic lncRNAs are transcribed between protein-coding genes and do not share promoters, exons or introns of protein-coding genes. lncRNAs have multiple functions including transcriptional activation and silencing of protein-coding genes, association with proteins to affect their function, and association with mRNAs to affect their translation and thus play essential roles in arrays of cellular processes [4] , [5] , [9] , [10] , [11] , [12] , [13] , [14] , [15] , [16] , [17] , [18] , [19] , [20] , [21] , [22] , [23] . Over or underexpression of lncRNAs is associated with various pathologic states in humans and animal models [23] , [24] , [25] , [26] , [27] . Differentiation of naïve T helper cells into effector T helper subsets including TH1, TH2 and TH17 selectively expressing cytokines, IFN-γ, IL-4, IL-5, IL-13 and IL-17, respectively, is a critical step to orchestrate the adaptive immune response to pathogens [28] . Key transcription factors governing these cell-fate decisions include T-bet (TH1), GATA3 (TH2) and ROR-γt and BATF (TH17) [29] , [30] , [31] , [32] . Additional transcription factors contribute to these cell-fate decisions. In part, these transcription factors orchestrate complex epigenetic alterations at these gene loci leading to the selective activation and silencing of genes encoding lineage-specific cytokines [28] , [33] , [34] . The lncRNA Tmevpg1, also named NeST, lncR- Ifng -3’ AS or IFNG -AS1, is specifically expressed by the TH1 subset by a T-bet-dependent mechanism and is necessary for the efficient transcription of Ifng by the TH1 subset [35] . Tmevpg1 associates with the WDR subunit of mixed-lineage leukaemia histone H3 Lys 4 (H3K4) methyltransferases to increase H3K4 methylation at the Ifng locus in CD8 T cells [25] . Tmevpg1 is required to confer resistance to lethal Salmonella enterica infection in mice thus establishing an essential role for this lncRNA in the host response to a bacterial pathogen. GATA3 -AS1 fulfils the definition of a divergent lncRNA and is transcribed in the opposite direction from GATA3 in both mouse and human genomes. Both GATA3 -AS1 and GATA3 are co-expressed in mouse and human TH2 cells [36] , [37] . TH2 responses have been clearly linked to both allergy and asthma and the expression of GATA3 -AS1 is induced by allergens in allergic subjects. Although the functions of GATA3 -AS1 are unknown, GATA3 -AS1 may play a role in allergic or asthmatic responses in humans. Recent studies have also begun to define the lncRNAs expressed by murine T lymphocytes at varying stages of development and differentiation [36] . These analyses identify numbers of lncRNAs expressed by T cells, identity of lncRNAs exhibiting lineage-specific expression and the underlying mechanisms to achieve lineage-specific lncRNA expression. They also expand the number of lncRNAs that exhibit critical immune functions in tissue culture and animal models. However, critical gaps in our knowledge of the function of lncRNAs in the immune system and in T lymphocytes still remain and we have attempted to address some of those here. To improve our understanding of lncRNA expression in T cells, we used whole-genome sequencing (RNA-seq) to identify lncRNAs expressed in human T cells and those that are selectively expressed in T cells differentiated under TH1-, TH2- or TH17-polarizing conditions. The majority of lineage-specific lncRNA genes are co-expressed with adjacent lineage-specific protein-coding genes. These lncRNAs are predominantly intragenic with co-expressed protein-coding genes and are transcribed in sense and antisense orientations with approximately equal frequencies. Genes encoding TH lineage-specific mRNAs are not randomly distributed across the genome but are highly enriched in genomic regions containing genes encoding TH lineage-specific lncRNAs. Our analyses also identify a cluster of antisense lncRNAs transcribed from the RAD50 locus that are co-expressed with IL4 , IL5 and IL13 genes under TH2-polarizing conditions. Depletion of these lncRNAs demonstrates their critical requirement for the expression of TH2 cytokines, IL-4, IL-5 and IL-13. Collectively, our analyses identify new lncRNAs expressed in a TH lineage-specific manner and identify one lncRNA cluster required for the expression of genes encoding TH2 cytokines. TH lineage-specific lncRNAs We performed whole-genome RNA sequencing (RNA-seq) to identify lncRNAs expressed in a TH1, TH2 or TH17 lineage-specific fashion by human T cells. RNA data were aligned with TopHat2 and RNA expression levels were quantified using Cufflinks [38] , [39] . Two examples of sequence assembly of known lncRNA/mRNA gene pairs, IFNG and TMEVPG1 (NEST, IFNG -AS1), and GATA3 and GATA3 -AS1, are shown in Supplementary Fig. 1 . Results from RNA-seq data were expressed as fragments per kilobase per million reads (FPKMs) determined using Cuffdiff. False discovery rates (<0.05) corrected for multiple testing. We annotated both mRNAs and lncRNAs using respective references from gencode.v17 (refs 40 , 41 ). To assess the quantitative accuracy of our RNA-seq analysis, we compared the expression levels from one individual of 34 protein-coding genes determined by RNA-seq and by quantitative RT–PCR [42] . We found that quantitative transcript determinations were highly correlated across this gene set that exhibited a wide expression range (>10 4 ; Supplementary Fig. 2a ). Thus, quantitation of transcript levels by RNA-seq yielded similar results to quantitative RT–PCR. Current estimates suggest that 20,000–25,000 protein-coding genes and about 10,000 lncRNA-coding genes exist in a human genome [2] . Of these, about 10,900 protein-coding genes and about 2,800 lncRNA-coding genes were expressed at detectable levels in our cultures (FPKM>1, Supplementary Fig. 2b , Supplementary Data 1 , expressed mRNA and expressed ncRNA sheets). Mean expression levels of all mRNAs were significantly higher than mean the expression levels of all lncRNAs (approximately threefold) as were median levels of mRNAs relative to lncRNAs ( Supplementary Fig. 2c ). Thus, similar to findings in other experimental systems, mean and median levels of all lncRNA transcripts were lower than mean and median levels of all the mRNA transcripts in peripheral blood mononuclear cell (PBMC) cultures. For further quality control, we assessed the expression levels of genes encoding TH lineage-specific cytokines and transcriptional regulators. IFNG was selectively expressed under TH1-polarizing conditions, IL4 , IL5 and IL13 were selectively expressed under TH2-polarizing conditions, and IL17F and IL10 were predominantly expressed under TH17-polarizing conditions in both primary and effector cultures ( Fig. 1a ). Key transcriptional regulators of TH1: TBX21 , TH2: GATA3 , and TH17: RORC and BATF , speciation were predominantly expressed in primary and effector TH1, TH2 and TH17 cultures, respectively. Thus, our culture conditions drove the selective expression of genes encoding lineage-specific cytokines and transcriptional regulators. 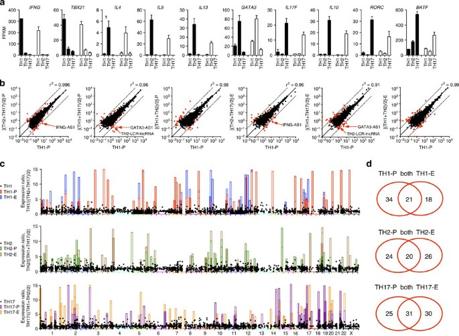Figure 1: Expression of genes encoding TH lineage-specific cytokines, known lineage-specific transcriptional regulators and lineage-specific lncRNAs determined by RNA-seq. (a) Expression of genes encoding lineage-specific cytokines and lineage-specific transcriptional regulators in primary (closed columns) and effector cultures (open columns).Results are expressed as normalized sequence reads in FPKM, fragments per kilobase of transcript per million mapped reads, error bars represent the range of data (n=2). (b) Scatterplots depicting expression levels of lncRNAs (FPKM) in specific primary and effector lineages (x-axes) relative to the alternative lineages (Y-axes), P denotes primary cultures, E denotes effector cultures. For example, thexaxis in the first graph shows FPKM levels for each lncRNA in primary TH1 cultures, TH1-P and theyaxis shows the average FPKM for each lncRNA in primary TH2 and TH17 cultures. The line was determined by Pearson’s linear regression,r2. The dashed lines depict one log above or below a slope of one. Red symbols denote lncRNAs differentially expressed by >fivefold between the two groups. The remaining graphs were calculated by the same method. (c) Modified ‘Manhattan’ plots to depict the distribution of expressed lncRNAs across the genome. Closed circles depict lncRNAs not differentially expressed in primary and effector TH cultures (<fourfold differences). Coloured open spikes depict lncRNAs selectively overexpressed (> fourfold differences in ratios) in the indicated primary and effector TH lineage cultures. (d) Venn diagrams tabulating numbers of lncRNAs overexpressed only in primary TH lineage cultures, only in effector TH lineage cultures or both primary and effector TH lineage cultures. Figure 1: Expression of genes encoding TH lineage-specific cytokines, known lineage-specific transcriptional regulators and lineage-specific lncRNAs determined by RNA-seq. ( a ) Expression of genes encoding lineage-specific cytokines and lineage-specific transcriptional regulators in primary (closed columns) and effector cultures (open columns).Results are expressed as normalized sequence reads in FPKM, fragments per kilobase of transcript per million mapped reads, error bars represent the range of data ( n =2). ( b ) Scatterplots depicting expression levels of lncRNAs (FPKM) in specific primary and effector lineages ( x -axes) relative to the alternative lineages (Y-axes), P denotes primary cultures, E denotes effector cultures. For example, the x axis in the first graph shows FPKM levels for each lncRNA in primary TH1 cultures, TH1-P and the y axis shows the average FPKM for each lncRNA in primary TH2 and TH17 cultures. The line was determined by Pearson’s linear regression, r 2 . The dashed lines depict one log above or below a slope of one. Red symbols denote lncRNAs differentially expressed by >fivefold between the two groups. The remaining graphs were calculated by the same method. ( c ) Modified ‘Manhattan’ plots to depict the distribution of expressed lncRNAs across the genome. Closed circles depict lncRNAs not differentially expressed in primary and effector TH cultures (<fourfold differences). Coloured open spikes depict lncRNAs selectively overexpressed (> fourfold differences in ratios) in the indicated primary and effector TH lineage cultures. ( d ) Venn diagrams tabulating numbers of lncRNAs overexpressed only in primary TH lineage cultures, only in effector TH lineage cultures or both primary and effector TH lineage cultures. Full size image To initiate the identification of human TH lineage-specific lncRNAs, we compared the expression levels in primary or effector cultures of one lineage, for example, TH1, TH2 and TH17, to the expression in the opposing cultures, for example, TH2 and TH17, TH1 and TH17, TH1 and TH2, respectively, using equations: (TH2 levels+TH17 levels/2and so on) resulting in a total of six comparisons. Data were analysed using scatterplots and linear regression. All six comparisons produced r 2 >0.9 indicating that most lncRNAs were not differentially expressed among different cell populations ( Fig. 1b ). lncRNAs with >5-fold differences in expression were identified by red symbols. IFNG-AS1, GATA3-AS1 and the novel TH2 locus control region (LCR) lncRNA were among these lineage-specific lncRNAs. Similar analyses of mRNAs were also performed ( Supplementary Fig. 3 ) and similar results were obtained. We next aligned the expressed lncRNAs to the genome (build hg19) to determine the genomic distributions of lineage-specific lncRNAs overexpressed in primary and/or effector cultures ( Fig. 1c ). Certain chromosomes, for example, 6, 13, were relatively devoid of lineage-specific lncRNAs. TH1 lineage-specific lncRNAs were enriched on chromosomes 12 and 17, TH2 lineage-specific lncRNAs were enriched on chromosomes 2 and 9, and TH17 lineage-specific lncRNAs were enriched on chromosomes 2, 16 and 17 (χ 2 , P <0.0001). These comparisons also more clearly identified those lncRNAs overexpressed in primary and/or effector cultures. Of >2,000 lncRNAs expressed in these T-cell cultures, only small percentages were TH lineage-specific lncRNAs. A Venn diagram was employed to illustrate this feature ( Fig. 1d ). Next, we identified those lncRNAs from the above analyses preferentially expressed in both primary and effector cultures in a lineage-specific manner. For example, mouse and human T cells selectively express IFNG -AS1 (TMEVPG1, NEST) under TH1-polarizing conditions and this was confirmed by our RNA-seq analysis ( Fig. 2a ). A novel lncRNA, AC007278.3, was also expressed in a TH1 lineage-specific manner. We identified a total of 34 lncRNAs selectively expressed in primary and effector TH1 cultures relative to primary and effector TH2 and TH17 cultures ( Supplementary Data 1 , TH1 ncRNA sheet). Mouse and human T cells selectively express GATA3 -AS1 under TH2-polarizing conditions [36] , [37] and this was confirmed by our RNA-seq analysis ( Fig. 2b ). Lineage-specific expression of IFNG -AS1 and GATA3 -AS1 was also confirmed by quantitative real-time PCR ( Supplementary Fig. 4 ). We identified a second novel lncRNA, TH2-LCR lncRNA, so named because the genomic position of this gene is located at the 3′ end of the RAD50 gene, the location of the previously described TH2-LCR in mice, and because it is selectively expressed in primary and effector TH2 cultures relative to primary and effector TH1 and TH17 cultures. In total, we identified 19 lncRNAs selectively expressed in primary and effector TH2 cultures relative to primary and effector TH1 and TH17 cultures ( Supplementary Data 1 , TH2 ncRNA sheet). The novel lncRNAs, RP11–98D18.3 and AC007182.6, were selectively expressed in primary and effector TH17 cultures relative to primary and effector TH1 and TH2 cultures ( Fig. 2c ). In total, we identified 26 lncRNAs exhibiting a similar lineage-specific expression pattern ( Supplementary Data 1 , TH17 ncRNA sheet). In contrast to the results reported for murine T cells [36] , we did not identify lncRNAs transcribed from genes adjacent to TBX21 or adjacent to genes encoding IL-17 cytokines using annotated lists. Overall, the majority of TH lineage-specific lncRNAs were expressed at higher levels in effector cultures (restimulation with anti-CD3) than in primary cultures (initial stimulation with anti-CD3 under TH1-, TH2- or TH17- polarizing conditions; heatmap, Fig. 2d ). This property was relatively uniform among TH1, TH2 and TH17 cultures. 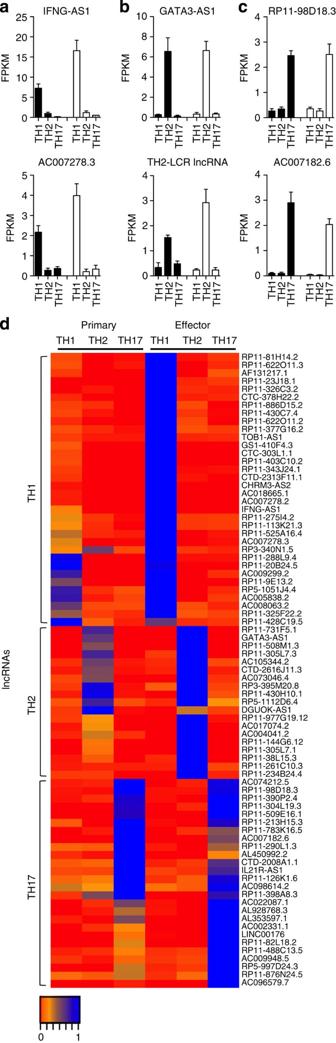Figure 2: Expression of T helper cell lineage-specific lncRNAs determined by RNA seq. (a–c) Expression levels of individual TH1, TH2 and TH17 lineage-specific lncRNAs, PBMC were cultured under TH1-, TH2- or TH17-polarizing conditions for 4 days (primary, filled columns). After 5 days, primary PBMC cultures were restimulated with plate-bound anti-CD3 for 2 days (effector, open columns) before harvest and analysis. Results are expressed as mean FPKM, error bars are s.d. determined by whole-genome RNA-seq (n=2). (d) A heatmap showing the expression levels of TH1, TH2 and TH17 lineage-specific lncRNAs derived from RNA-seq data. A scale bar is shown below the heatmap. Figure 2: Expression of T helper cell lineage-specific lncRNAs determined by RNA seq. ( a – c ) Expression levels of individual TH1, TH2 and TH17 lineage-specific lncRNAs, PBMC were cultured under TH1-, TH2- or TH17-polarizing conditions for 4 days (primary, filled columns). After 5 days, primary PBMC cultures were restimulated with plate-bound anti-CD3 for 2 days (effector, open columns) before harvest and analysis. Results are expressed as mean FPKM, error bars are s.d. determined by whole-genome RNA-seq ( n =2). ( d ) A heatmap showing the expression levels of TH1, TH2 and TH17 lineage-specific lncRNAs derived from RNA-seq data. A scale bar is shown below the heatmap. Full size image Co-expressed lncRNAs and mRNAs One function of lncRNAs is to regulate the expression of neighbouring protein-coding genes in the genome. For example, IFNG -AS1 and IFNG are co-expressed under TH1 culture conditions and IFNG -AS1 is required for IFNG transcription in both tissue culture and infectious models [25] , [35] . GATA3 and GATA3 -AS1 are co-expressed under TH2 culture conditions. To explore to what degree this general notion may be applied to TH lineage-specific lncRNAs, we identified TH lineage-specific mRNAs by calculating the expression level of individual mRNAs in one lineage versus the other two lineages using the ratios: expression in TH1/((expression in TH2+TH17)/2) and so forth. We aligned the genomic positions of genes encoding these mRNAs to genomic positions of genes encoding TH lineage-specific lncRNAs identified above. This genome-wide view demonstrated that genomic positions of TH lineage-specific protein-coding genes aligned with TH lineage-specific lncRNA-coding genes in many but not all instances ( Fig. 3 , Supplementary Data 1 ). 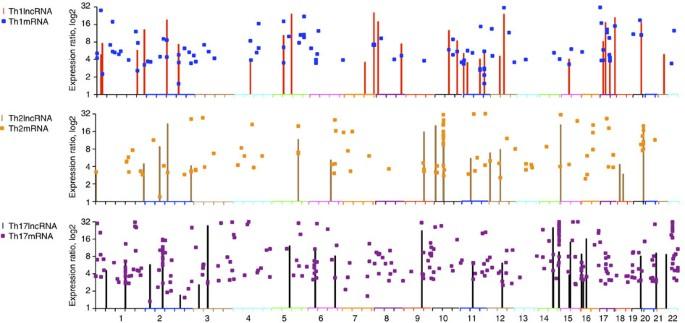Figure 3: Comparison between genomic locations of TH lineage-specific lncRNAs and mRNAs. xaxis depicts genomic positions according to chromosome and base pairs from p terminus (left) to q terminus (right) in kilobases. Theyaxis depicts the expression ratio, log2, of TH lineage-specific lncRNAs (spikes) and mRNAs (closed symbols). Expression ratios of each lncRNA and mRNA were determined by dividing FPKM for each lncRNA or mRNA determined in one TH lineage culture by the average FPKM determined in the combined other two TH lineage cultures. For example, TH1: FPKMTH1/((FPKMTH2+FPKMTH17)/2). Figure 3: Comparison between genomic locations of TH lineage-specific lncRNAs and mRNAs. x axis depicts genomic positions according to chromosome and base pairs from p terminus (left) to q terminus (right) in kilobases. The y axis depicts the expression ratio, log2, of TH lineage-specific lncRNAs (spikes) and mRNAs (closed symbols). Expression ratios of each lncRNA and mRNA were determined by dividing FPKM for each lncRNA or mRNA determined in one TH lineage culture by the average FPKM determined in the combined other two TH lineage cultures. For example, TH1: FPKM TH1 /((FPKM TH2 +FPKM TH17 )/2). Full size image To explore this possibility further, we determined the extent to which TH lineage-specific lncRNAs were co-expressed with nearby protein-coding genes in the genome. We identified nearby protein-coding genes within 150 kb of a TH lineage-specific lncRNA gene using the UCSC genome browser and employed Pearson’s linear regression to quantify co-expression across primary and effector TH1, TH2 and TH17 cultures. This analysis confirmed that IFNG -AS1 and IFNG were co-expressed and that GATA3 -AS1 and GATA3 were co-expressed in T-cell cultures ( Table 1 , see also Supplementary Table 1 for complete analysis to identify co-expressed lncRNA-mRNA pairs). We also found that the novel TH2-LCR lncRNA (AC004041.2) was co-expressed with IL4 , IL5 and IL13 genes. The TH2-LCR lncRNA-coding gene is located within RAD50 but was not co-expressed with RAD50 . We also found that the lncRNAs, RP11–98D18.3 and AC007182.6, were co-expressed with adjacent or nearby RORC and BATF genes, respectively. These results are consistent with the general notion that lncRNAs tend to regulate the nearby protein-coding genes and identified co-expressed protein-coding genes as potential lncRNA targets. However, it is relevant to note that our analysis extended across genomic regions of ∼ 300 kb containing multiple protein-coding genes compared with previous studies where much smaller genomic regions were analysed [6] . Table 1 TH lineage-specific lncRNAs are co-expressed with neighbouring protein-coding genes. Full size table We also identified lncRNAs with selectively reduced levels of expression in TH1, TH2 or TH17 culture conditions relative to opposing culture conditions, respectively. For example, we identified lncRNAs expressed at low levels in TH2 cultures and high levels in TH1 and TH17 cultures ( Supplementary Table 1 ). Like the lncRNAs, nearby co-expressed protein-coding genes were also uniformly underexpressed in TH2 cultures compared with TH1 and TH17 cultures. We also did not find negative correlations between the expression of lineage-specific lncRNAs and neighbouring protein-coding genes. Thus, these data do not support the concept that these lncRNAs may repress the transcription of neighbouring protein-coding genes. To further evaluate these points we compared the distances in kb between lineage-specific lncRNA genes and nearby co-expressed protein-coding genes and as a function of the number of protein-coding genes between lineage-specific lncRNA genes and of the adjacent co-expressed protein-coding genes in the genome. Both types of comparisons demonstrated that the majority of lineage-specific lncRNAs genes were intragenic with co-expressed protein-coding genes (85%) ( Fig. 4a,b ). Approximately 50% of protein-coding genes within 50 kb of a lineage-specific lincRNA gene or adjacent to a lineage-specific lincRNA gene were also co-expressed with the respective lncRNA gene. This frequency decreased by moving farther away from the genomic position of the lineage-specific lincRNA gene. Thus, proximity in the genome was an important contributor to whether or not protein-coding genes and lncRNA genes were co-expressed. We also asked if lncRNA genes were transcribed in the same (sense) or opposite (antisense) orientations to co-expressed protein-coding genes. We found that there was about a 50:50 distribution between lncRNA genes and co-expressed protein-coding genes transcribed from the same or opposite DNA strand ( Fig. 4c ). Thus, there was not a bias for lncRNA genes and co-expressed protein-coding genes to be transcribed from the same or opposite DNA strand. These results may seem contrary to the general notion that lncRNA/mRNA gene pairs tend to be transcribed divergently from the opposite DNA strands [5] , [6] . However, our analysis examined co-expressed lncRNA and protein-coding genes spanning a genomic distance of 300 kb. To further illustrate this point, we determined the number of co-expressed protein-coding genes within 150-kb upstream or downstream of a TH lineage-specific lncRNA gene. The majority of these clusters ( ∼ 85%) contained one or more co-expressed protein-coding genes ( Fig. 4d ). Approximately 30% of the clusters contained two or more co-expressed protein-coding genes and ∼ 15% of the clusters contained three or more co-expressed protein-coding genes. Thus, many TH lineage-specific protein-coding genes were positioned nearby lineage-specific lncRNA genes in the human genome. 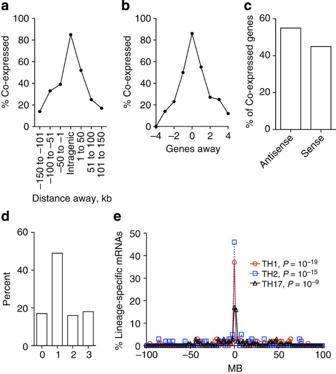Figure 4: Relationships between lineage-specific lncRNAs and co-expressed protein-coding genes. (a) Results are expressed as the % of protein-coding genes co-expressed with lineage-specific lncRNAs relative to total genes within the indicated distance from the lineage-specific lncRNA as a function of distance from the lncRNA in kilobases. (b) As inaexcept results are expressed relative to the number of genes in the genome away from the lineage-specific lncRNA. (c) Percentage of co-expressed genes transcribed in the antisense or sense orientation relative to the adjacent lncRNA. (d) Percentage of lncRNA-protein-coding gene lineage-specific clusters containing the indicated numbers of co-expressed protein-coding genes. See alsoSupplementary Table 1. (e) Genes encoding lineage-specific mRNAs are enriched in the genome within lineage-specific lncRNA gene clusters. Theyaxis is the percent of total lineage-specific (TH1, TH2 and TH17) mRNAs defined as threefold overexpressed in TH1, TH2 or TH17 cultures relative to the other two lineages. Thexaxis is the distance of the gene encoding a TH1-, TH2- or TH17-specific mRNA from the nearest gene encoding a TH1-, TH2- or TH17-specific lncRNA.Pvalues determined by χ2analysis. Figure 4: Relationships between lineage-specific lncRNAs and co-expressed protein-coding genes. ( a ) Results are expressed as the % of protein-coding genes co-expressed with lineage-specific lncRNAs relative to total genes within the indicated distance from the lineage-specific lncRNA as a function of distance from the lncRNA in kilobases. ( b ) As in a except results are expressed relative to the number of genes in the genome away from the lineage-specific lncRNA. ( c ) Percentage of co-expressed genes transcribed in the antisense or sense orientation relative to the adjacent lncRNA. ( d ) Percentage of lncRNA-protein-coding gene lineage-specific clusters containing the indicated numbers of co-expressed protein-coding genes. See also Supplementary Table 1 . ( e ) Genes encoding lineage-specific mRNAs are enriched in the genome within lineage-specific lncRNA gene clusters. The y axis is the percent of total lineage-specific (TH1, TH2 and TH17) mRNAs defined as threefold overexpressed in TH1, TH2 or TH17 cultures relative to the other two lineages. The x axis is the distance of the gene encoding a TH1-, TH2- or TH17-specific mRNA from the nearest gene encoding a TH1-, TH2- or TH17-specific lncRNA. P values determined by χ 2 analysis. Full size image A second means we employed to explore the relationship between lineage-specific mRNA genes and lineage-specific lncRNA genes was to identify positions in the genome of genes encoding lineage-specific mRNAs and genes encoding lineage-specific lncRNAs ( Supplementary Data 1 ). We defined an mRNA as a lineage-specific mRNA gene if its expression level in one lineage, for example, TH1, was threefold over the expression level in the other two lineages, for example, TH2, TH17, in both primary and effector cultures. This analysis identified 105 TH1-specific mRNA genes, 110 TH2-specific mRNA genes and 327 TH17-specific mRNA genes. The high number of TH17-specific mRNAs was due, in part to the TH17-specific expression of many Ig variable region gene segments on chromosomes 14 and 22 and these were included in the analysis. We next determined the distance of genes encoding TH1, TH2 and TH17 lineage-specific mRNAs in the genome from adjacent genes encoding TH1, TH2 and TH17 lineage-specific lncRNAs using the UCSC genome browser (hg19; 2009 build). Our rationale was that this would allow us to determine if genes encoding lineage-specific mRNAs were randomly distributed across the genome or were close to a lineage-specific lncRNA gene. We found that 37, 46 and 17% of genes encoding TH1, TH2 or TH17 lineage-specific mRNAs were within 300 kb of a gene encoding a TH1, TH2,or TH17 lineage-specific lncRNA ( Fig. 4e ). We interpreted these results to indicate that genes encoding lineage-specific mRNAs are enriched in the genome in regions containing genes encoding lineage-specific lncRNAs and are not randomly distributed across the genome ( P =10 −19 , 10 −15 and 10 −9 ; TH1, TH2 and TH17, respectively, χ 2 analysis). TH2 cytokines are regulated by the TH2-LCR lncRNA cluster Inspection of the UCSC genome browser revealed that the TH2-LCR lncRNA, consisted of as many as four alternatively spliced transcripts ( Fig. 5a ). We compared these RNA sequences and found that each transcript contained a shared sequence of ∼ 100 bp ( Fig. 5b , green). The orange partial sequence was also shared but the partial sequences were of two lengths. A third partial sequence was shared by three transcripts (red) and a fourth partial sequence was shared by two transcripts (blue). Partial sequences in black were unique for each transcript and not shared ( Supplementary Fig. 5 ). We designed PCR primer pairs unique to each alternatively spliced transcript to determine TH2 lineage-specific expression patterns. We found that each alternatively spliced transcript (labelled 1–4) was selectively expressed in TH2 cultures relative to TH1 and TH17 cultures ( Fig. 5c ). We designed a small interfering RNA (siRNA) to the 100-bp sequence shared by all the transcripts (green, Fig. 5b ) to deplete all the four TH2-LCR lncRNA alternatively spliced transcripts in the TH2 cultures. This siRNA did not target a RAD50 exon ( Supplementary Fig. 6a ). We performed intracellular cytokine staining to quantify IL-4, IL-5 and IL-13 expression after the transfection of developing TH2 cells with either a control siRNA or this specific siRNA. We found that the siRNA designed to target all TH2-LCR lncRNA alternatively spliced transcripts resulted in profound loss of IL-4, IL-5 and IL-13 expression by TH2 cultures ( Fig. 5d , see also Supplementary Fig. 6b ). In contrast, transfection with this siRNA did not alter the total cell numbers or cell apoptosis as measured by flow cytometry using annexin V and 7-AAD ( Supplementary Fig. 7a–c ). Thus, these results demonstrate that these TH2 lineage-specific lncRNAs are required for the efficient expression of each of the adjacent genes encoding TH2 cytokines, IL-13, IL-4 and IL-5, at least under these culture conditions, which is a measure of TH2 lineage commitment or TH2 differentiation. 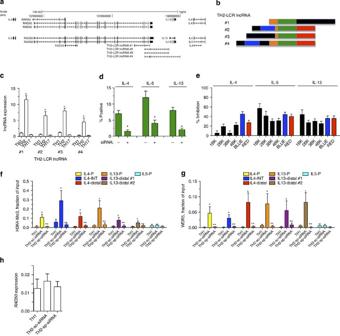Figure 5: TH2-LCR lncRNA regulates IL-4, IL-5 and IL-13 expression. (a) Genomic organization ofIL5,RAD50,IL13andIL4and the TH2-LCR lncRNA cluster (UCSC genome browser). (b) Shared and unique RNA sequences in alternatively spliced TH2-LCR lncRNAs. Black: non-shared sequences, green: shared sequences among all TH2-LCR lncRNAs, red: identify shared by three lncRNAs, orange; long and short sequence identity shared by all or two transcripts, blue: sequence identity shared by two transcripts. (c) TH2-LCR lncRNA transcripts are TH2 lineage-specific. PCR primers were designed to detect each TH2-LCR lncRNA alternatively spliced transcript by RT–PCR. Results are mean expression±s.d. after normalization toGAPDH(n=4). *P<0.05 in TH2 versus TH1 and TH17 cultures. (d) Depletion of TH2-LCR lncRNA abrogates IL-4, IL-13 and IL-5 expression by TH2 cells. TH2 cultures were transfected with a negative control siRNA (−) or siRNA (+) targeting the TH2-LCR lncRNA shared sequence (green,b). Intracellular cytokine staining was performed. Results are expressed as mean % CD4+ T cells expressing each cytokine±s.d. (n=4). *P<0.05 comparing transfections with control siRNA to TH2-LCR lncRNA-specific siRNA. (e) Effect of siRNA-mediated knockdown of individual TH2-LCR lncRNA transcripts on IL-4, IL-13 and IL-5 expression by TH2 cells. siRNAs were designed to target individual TH2-LCR lncRNAs, BK1, BK2, BK3, BK4, two TH2-LCR lncRNAs (blue) or three TH2-LCR lncRNAs (red; seeb). IL-4, IL-13 and IL-5 expression was determined by intracellular cytokine staining. Results are expressed as % inhibition relative to transfection with scrambled siRNA control±s.d. (n=3). (f,g) Effects of TH2-LCR lncRNA knockdown on formation of H3K4-Me3 marks (f) and WDR5 localization (g) atIL4,IL13andIL5loci. Non-transfected TH1 cultures and TH2 cultures, transfected with a scrambled siRNA (TH2-sc-siRNA) or TH2-LCR lncRNA-specific siRNA (TH2-sp-siRNA) on day 3, were harvested on day 5. Levels of H3K4-Me3 or WDR5 were determined by ChIP and are expressed as a fraction of input±s.d. (n=3). *P<0.05 comparing either TH1 to TH2-sc-RNA cultures or **TH2-sc-siRNA to TH2-sp-siRNA cultures. (h) Effect of TH2-LCR lncRNA knockdown onRAD50expression. As ind, except RNA was isolated andRAD50transcript levels±s.d. determined after normalization toGAPDH(n=3).Pvalues were determined using Student’st-test. Figure 5: TH2-LCR lncRNA regulates IL-4, IL-5 and IL-13 expression. ( a ) Genomic organization of IL5 , RAD50 , IL13 and IL4 and the TH2-LCR lncRNA cluster (UCSC genome browser). ( b ) Shared and unique RNA sequences in alternatively spliced TH2-LCR lncRNAs. Black: non-shared sequences, green: shared sequences among all TH2-LCR lncRNAs, red: identify shared by three lncRNAs, orange; long and short sequence identity shared by all or two transcripts, blue: sequence identity shared by two transcripts. ( c ) TH2-LCR lncRNA transcripts are TH2 lineage-specific. PCR primers were designed to detect each TH2-LCR lncRNA alternatively spliced transcript by RT–PCR. Results are mean expression±s.d. after normalization to GAPDH ( n =4). * P <0.05 in TH2 versus TH1 and TH17 cultures. ( d ) Depletion of TH2-LCR lncRNA abrogates IL-4, IL-13 and IL-5 expression by TH2 cells. TH2 cultures were transfected with a negative control siRNA (−) or siRNA (+) targeting the TH2-LCR lncRNA shared sequence (green, b ). Intracellular cytokine staining was performed. Results are expressed as mean % CD4+ T cells expressing each cytokine±s.d. ( n =4). * P <0.05 comparing transfections with control siRNA to TH2-LCR lncRNA-specific siRNA. ( e ) Effect of siRNA-mediated knockdown of individual TH2-LCR lncRNA transcripts on IL-4, IL-13 and IL-5 expression by TH2 cells. siRNAs were designed to target individual TH2-LCR lncRNAs, BK1, BK2, BK3, BK4, two TH2-LCR lncRNAs (blue) or three TH2-LCR lncRNAs (red; see b ). IL-4, IL-13 and IL-5 expression was determined by intracellular cytokine staining. Results are expressed as % inhibition relative to transfection with scrambled siRNA control±s.d. ( n =3). ( f , g ) Effects of TH2-LCR lncRNA knockdown on formation of H3K4-Me3 marks ( f ) and WDR5 localization ( g ) at IL4 , IL13 and IL5 loci. Non-transfected TH1 cultures and TH2 cultures, transfected with a scrambled siRNA (TH2-sc-siRNA) or TH2-LCR lncRNA-specific siRNA (TH2-sp-siRNA) on day 3, were harvested on day 5. Levels of H3K4-Me3 or WDR5 were determined by ChIP and are expressed as a fraction of input±s.d. ( n =3). * P <0.05 comparing either TH1 to TH2-sc-RNA cultures or **TH2-sc-siRNA to TH2-sp-siRNA cultures. ( h ) Effect of TH2-LCR lncRNA knockdown on RAD50 expression. As in d , except RNA was isolated and RAD50 transcript levels±s.d. determined after normalization to GAPDH ( n =3). P values were determined using Student’s t -test. Full size image To further explore the relationship among alternatively spliced TH2-LCR lncRNAs and regulation of TH2 cytokine expression, we tested siRNAs that selectively targeted each individual alternatively spliced lncRNA transcript, two of the four alternatively spliced lncRNA transcripts, or three of the four alternatively spliced transcripts. We reasoned that this would help distinguish between the possibilities that individual lncRNA alternatively spliced transcripts are required for the expression of individual cytokines, IL-13, IL-4 or IL-5, or that individual lncRNA alternatively spliced transcripts cooperate to induce IL-13, IL-4 and IL-5 expression. We stimulated human PBMC with anti-CD3 under TH2-polarizing conditions. We transfected either a scrambled siRNA or siRNAs that targeted individual siRNAs, designated BK1, BK2, BK3 and BK4 ( Fig. 5b ) or targeted a sequence shared by two lncRNAs (blue, Fig. 5b ) or shared by three alternatively spliced lncRNA transcripts (red, Fig. 5b ). Transfection of each siRNA resulted in the efficient loss of target TH2-LCR lncRNA transcripts ( Supplementary Fig. 6b–e ). We expressed our results as % inhibition of cytokine expression determined by flow cytometry relative to scrambled siRNA. We did not find that the knockdown of one alternatively spliced lncRNA, for example, BK1, resulted in the selective loss of expression of one TH2 cytokine, for example, IL-4, and that the knockdown of a second alternatively spliced lncRNA, for example, BK2, resulted in the selective loss of expression of a second TH2 cytokine, for example, IL-13 and so on ( Fig. 5e ). Rather, we found partial inhibition of IL-4, IL-5 or IL-13 cytokine expression by targeting individual alternatively spliced TH2-LCR lncRNAs via siRNA knockdown but this inhibition was not as great as the degree of inhibition observed by siRNA targeted knockdown of all TH2-LCR lncRNA alternatively spliced isoforms (compare Fig. 5d with Fig. 5e ). Our conclusion is that alternatively spliced lncRNAs function cooperatively to drive TH2 cytokine expression. Further experimentation will be required to determine the underlying mechanisms by which alternatively spliced lncRNAs function to stimulate IL-4, IL-5 and IL-13 expression. In murine T cells, the TH2-LCR is necessary to establish histone H3K4Me marks at Il4 , Il13 and Il5 promoters and distal DNA regulatory elements surrounding these genes. One function of lncRNAs is to recruit the enzymes required to produce H3K4Me marks to the genomic loci. Therefore, we reasoned that the TH2-LCR lncRNA may be required to establish H3K4Me marks at IL4 , IL5 and IL13 promoters and distal regulatory elements. We first asked if TH2-LCR lncRNA was preferentially localized to either cytoplasmic or nuclear fractions in TH2-polarized cells. We found that each TH2-LCR lncRNA transcript was enriched in the nuclear fraction ( Supplementary Fig. 8 ). To further explore this hypothesis, we transfected scrambled control siRNA or TH2-LCR lncRNA-specific siRNA to knockdown all TH2-LCR lncRNA transcripts and performed chromatin immunoprecipitation (ChIP) assays to quantify the levels of H3K4Me3 marks at these promoters and distal conserved DNA sequences. We determined the levels of H3K4Me3 in primary TH1 cells (negative control), primary TH2 cells transfected with a nonspecific scrambled siRNA (positive control) and primary TH2 cells transfected with the siRNA specific for TH2-LCR lncRNA. H3K4Me3 marks at different genomic positions we analysed were very low in TH1 cells compared with TH2 cells ( Fig. 5f ). Knockdown of the TH2-LCR lncRNA resulted in a marked decrease in H3K4Me3 at the IL4 promoter, IL4 intron and an IL4 distal conserved region and the IL13 promoter, and one IL13 distal conserved element. In contrast, we did not detect the loss of H3K4Me3 marks at a second IL13 distal conserved element after siRNA treatment even though we detected TH2-dependent enrichment of H3K4Me3 marks at this distal conserved element. We also did not detect the enrichment of H3K4Me3 at the IL5 promoter in TH2-polarized cells. Nevertheless, we conclude that one function of the TH2-LCR lncRNA is to facilitate the formation of H3K4Me3 marks at multiple genomic positions at IL4 and IL13 loci. At this point our analysis cannot exclude the possibility that TH2-LCR lncRNA is required for H3K4 methylation at other sites spanning the IL5 genomic locus and further investigations will be required to evaluate this question. We performed a second series of ChIP assays at IL4 , IL5 and IL13 promoters and distal regulatory elements in TH1 cells and TH2 cells transfected with a nonspecific scrambled siRNA or siRNA specific for TH2-LCR lncRNA and quantified levels of WDR5 bound to promoters and distal sequences ( Fig. 5g ). Recruitment of WDR5 to these genomic regions was very low in TH1 cultures compared with TH2 cultures treated with scrambled siRNA. However, treatment with the siRNA specific for the TH2-LCR lncRNA reduced WDR5 recruitment to the IL4 promoter, IL4 intron and IL4 distal sequence along with the IL13 promoter and two IL13 distal regulatory elements. Similar to what we observed with the H3K4Me3 marks, we did not find any change in WDR5 recruitment to the IL5 promoter. We interpret these results to indicate that TH2-LCR lncRNAs recruit WDR5-containing complexes to these regulatory genomic elements. As an additional experimental comparator, we examined the expression levels of RAD50 in TH2 cells transfected with the scrambled siRNA or the TH2-LCR lncRNA-specific siRNA. Transfection of the TH2-LCR lncRNA siRNA did not alter the expression levels of RAD50 ( Fig. 5h ). Lineage-specific lncRNAs bind to hnRNPs and WDR5 Two general classes of nuclear proteins that lncRNAs associate with are the heterogeneous nuclear ribonucleoproteins (hnRNPs) and components of the H3K4 methyltransferase protein complex [5] , [16] , [18] . To initiate studies to explore the association of TH lineage-specific lncRNAs with these protein complexes we performed immunoprecipitation using either an isotype control antibody, a pan hnRNP antibody that recognizes over 10 hnRNPs or an antibody against WDR5, a component of the histone H3K4 methyltransferase complex and determined the recovery of lncRNAs in immunoprecipitates. These analyses showed specific pull-down of pan hnRNP and WDR5 by immunoprecipitation ( Supplementary Fig. 9 ) and that TH2-LCR lncRNA associated with hnRNPs and WDR5 ( Fig. 6 ). IFNG -AS1 also associated with both hnRNPs and WDR5. Previous analyses using somewhat different methodology demonstrated that IFNG -AS1 associates with WDR5 (ref. 25 ). In contrast, GATA3 -AS1 did not associate with either hnRNP or WDR5, suggesting other modes of action. As a control, we determined that GAPDH mRNA transcripts did not associate with hnRNPs or WDR5. Overall, this may prove a useful means to classify TH lineage-specific lncRNAs but will require significantly greater analyses than that performed here. 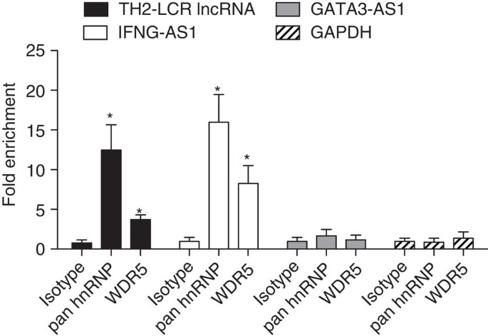Figure 6: TH lineage-specific lncRNAs associate with hnRNPs and WDR5. Whole-cell lysates were prepared from TH1 and TH2 cultures and incubated with either an isotype Ig control antibody (isotype), a pan hnRNP antibody (recognizes a conserved hnRNP amino acid sequence) or a WDR5 antibody. Immunoprecipitates were harvested with protein A/G sepharose beads, RNA was isolated and the lncRNA transcripts in the immunoprecipitates were determined by quantitative PCR. Fold enrichment±s.d. (n=3) was determined by comparing the specific Ct obtained from the isotype immunoprecipitate to the antibody-specific immunoprecipitate by calculating 2(IsotypeCt-Ab-specificCt). *=P<0.05 determined using Student’st-test. Figure 6: TH lineage-specific lncRNAs associate with hnRNPs and WDR5. Whole-cell lysates were prepared from TH1 and TH2 cultures and incubated with either an isotype Ig control antibody (isotype), a pan hnRNP antibody (recognizes a conserved hnRNP amino acid sequence) or a WDR5 antibody. Immunoprecipitates were harvested with protein A/G sepharose beads, RNA was isolated and the lncRNA transcripts in the immunoprecipitates were determined by quantitative PCR. Fold enrichment±s.d. ( n =3) was determined by comparing the specific Ct obtained from the isotype immunoprecipitate to the antibody-specific immunoprecipitate by calculating 2 (IsotypeCt-Ab-specificCt) . *= P <0.05 determined using Student’s t -test. Full size image De novo analysis of TH lineage-specific lincRNAs Finally, we sought to identify novel transcripts from our polarized T-cell cultures by performing a de novo transcript assembly using Cufflinks following previously established methodologies (see Methods and Supplementary Fig. 10 ). We identified 305,095 novel transcripts and applied filters to remove known protein-coding and noncoding annotated genes and novel transcripts that exhibited protein-coding potential. From these analyses, we identified 28 TH1, 17 TH2 and 29 TH17 lineage-specific lincRNA transcripts expressed at >1 FPKM in primary or effector cultures and exhibiting >5-fold expression differences compared with the other polarized cultures ( Fig. 7a , Supplementary Fig. 10 , and Supplementary Data 1 ). One concern from our de novo transcript assembly was the likelihood of identifying unannotated neighbouring protein-coding gene extensions, a technical concern noted by others attempting to identify novel lncRNA transcripts across [1] , [43] . Thus, we excluded from our analysis transcripts exhibiting any overlap with protein-coding genes and have identified only long intergenic noncoding RNAs. These lineage- specific novel lncRNA transcripts were expressed at greater levels in effector than primary TH1, TH2 and TH17 cultures, respectively ( Fig. 7b ). We used the Integrated Genome Browser and the UCSC Genome Browser to identify nearby protein-coding genes and Pearson’s linear regression to quantify co-expression. From these analyses, 43, 41 and 52% of TH1, TH2 and TH17 lineage-specific novel lincRNA transcripts were co-expressed with nearby protein-coding genes ( Fig. 7c ). This was very similar to what we observed in our analysis of annotated lncRNAs. These locations are likely to be incomplete due to the computational limitations in transcript assembly from RNA-seq data and some annotations could overlap and form larger lincRNA transcripts. Additional studies are required to validate these novel lincRNAs in primary human samples and to define independent, complete lincRNA transcript annotations [43] . 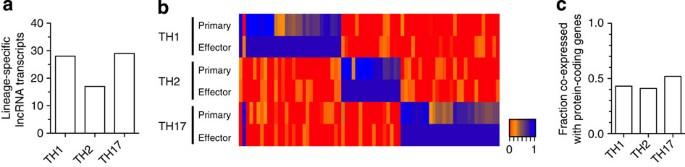Figure 7: Discovery of novel TH lineage-specific lincRNAs. (a) Numbers of lineage-specific novel lincRNAs were identified throughde novoassembly of transcripts from whole-genome RNA-sequencing data followed by a series of filters removing known and novel protein-coding transcripts and noncoding RNAs <200 bp in length. Identified novel lineage-specific lincRNAs are expressed >1 FPKM in either the primary or effector culture (see also Methods andSupplementary Fig. 10). (b) Heatmap data showing levels of lineage-specific novel lincRNA expression by primary and effector TH1, TH2 and TH17 cultures. (c) Co-expression of novel lincRNAs with neighbouring protein-coding genes expressed as the fraction of identified lineage-specific TH1, TH2 or TH17 lincRNAs co-expressed with protein-coding genes within 250 kb 5′ or 3′ of the given lncRNA gene. Figure 7: Discovery of novel TH lineage-specific lincRNAs. ( a ) Numbers of lineage-specific novel lincRNAs were identified through de novo assembly of transcripts from whole-genome RNA-sequencing data followed by a series of filters removing known and novel protein-coding transcripts and noncoding RNAs <200 bp in length. Identified novel lineage-specific lincRNAs are expressed >1 FPKM in either the primary or effector culture (see also Methods and Supplementary Fig. 10 ). ( b ) Heatmap data showing levels of lineage-specific novel lincRNA expression by primary and effector TH1, TH2 and TH17 cultures. ( c ) Co-expression of novel lincRNAs with neighbouring protein-coding genes expressed as the fraction of identified lineage-specific TH1, TH2 or TH17 lincRNAs co-expressed with protein-coding genes within 250 kb 5′ or 3′ of the given lncRNA gene. Full size image An abundance of lncRNA genes are present in eukaryotic genomes. The full scope of their transcriptional regulation and functions is only beginning to be understood. The purposes of the studies described here were to (a) employ whole-genome RNA-seq to determine the scope of TH lineage-specific lncRNA expression, (b) explore the relationships between the genes encoding TH lineage-specific lncRNAs and the TH lineage-specific mRNAs and (c) define new functions of TH lineage-specific lncRNAs. Whole-genome RNA-seq reveals numerous lncRNAs selectively expressed under TH1-, TH2- and TH17-polarizing conditions. Several of these, IFNG -AS1 (NeST, TMEVPG1) and GATA3 -AS1, are known to exhibit selective expression under TH1 or TH2-polarizing conditions. Their genomic positions and this response are conserved between mouse and human lymphocytes. Others appear novel. A common feature of these lncRNAs is that they tend to be co-expressed with intragenic or adjacent protein-coding genes. As such, these results may suggest that these lncRNAs are potential positive regulators of these intragenic or adjacent co-expressed protein-coding genes. However, this needs to be determined experimentally. There is not a clear preference for transcription of TH-specific lncRNAs and co-expressed protein-coding genes to be in the antisense orientation, which is, for example, a feature of IFNG and IFNG -AS1, and GATA3 and GATA3 -AS1. Rather, about half of TH-specific lncRNAs and their co-localized and co-expressed protein-coding genes are transcribed from the same DNA strand and about half are transcribed from the opposite DNA strand. Similarly, in the mouse, the lncRNA, lincR- Ccr2 -5’AS, regulates expression of adjacent Ccr1 (sense) and Ccr3 (antisense), Ccr2 (antisense) and Ccr5 (antisense) genes [36] . In the case of TH2-LCR lncRNA, these lncRNA isoforms are transcribed antisense to IL4 and IL13 but sense to IL5 . Thus, besides being co-expressed, these lncRNAs contribute to the transcription of neighbouring functionally related genes oriented in both the sense and antisense direction in relationship with the respective lncRNA genes. The majority of TH-specific lncRNAs are co-expressed with a neighbouring protein-coding gene. In fact many, >30% are co-expressed with two or more neighbouring protein-coding genes. The majority of these co-expressed genes encode proteins with immunologic functions. Our work may also allow for the discovery of lncRNAs that can be translated into basic research programs utilizing murine models to study the functions of these lncRNAs in greater detail. There are examples of mouse lncRNAs that are syntenic orthologues of human lncRNAs. Noteworthy examples are Ifng-AS1 (human: IFNG -AS1) and Gata3-AS1 (human: GATA3 -AS1), which we report in our current work studying human polarized TH1 and TH2 cultures and that were previously reported in genome-wide profiling studies of lincRNAs in murine Th1- and Th2-polarized cells [36] . Our preliminary analysis combining bioinformatic and visual inspection of identified lineage-specific transcripts in humans. suggests that only a small percentage of identified human TH lineage-specific lncRNAs are also observed in murine systems. This observation is corroborated by findings published elsewhere, directly comparing human and mouse lncRNA conservation, which found that ∼ 15% of lncRNAs identified in human primary samples were expressed in mice [44] . These analyses further highlight the lack of conservation of these noncoding elements across mammalian genomes. For example, in the mouse, TH lineage-specific lncRNAs exist adjacent to both Tbx21 and the Il17 family of genes [36] . In the human genome, lncRNA genes exist in close proximity to TBX21 and the IL17 family of genes. However, these are not expressed in a TH-specific fashion. Multiple functions of lncRNAs have been described. Results presented here serve as a resource for future investigations to identify the functions of these novel TH-specific lncRNAs. One such group of novel TH-specific lncRNAs is the TH2-LCR lncRNA cluster consisting of four unique transcripts. Each has a unique transcriptional start site and shares one RAD50 exon plus RAD50 intronic sequences in the lncRNA transcript. Three lncRNAs share a second RAD50 exon plus additional RAD50 intronic sequences. All four alternatively spliced lncRNAs are TH2 lineage-specific and co-expressed with IL4 , IL5 and IL13 but not RAD50 . Thus, they partially fit the definition of an antisense lncRNA with RAD50 representing the protein-coding gene. Depletion of the TH2-LCR lncRNA by using siRNA targeting the ∼ 100-bp shared sequence demonstrates that it is necessary for the expression of genes encoding TH2 cytokines, IL-4, IL-5 and IL-13. This same genomic region in the mouse has been defined as a TH2-LCR, which is required for expression of genes encoding TH2 cytokines, in vitro and in vivo , and for the pathogenesis of allergic asthma [27] , [45] . In general, LCRs are functionally defined as genomic elements required for the expression and silencing of linked genes, usually a gene family such as developmentally regulated globin genes or lineage-specific genes encoding the TH2 family of cytokines. Exactly how these LCRs function to activate or silence these families of genes is not completely understood [46] , [47] . Our results are consistent with the notion that one mechanism by which LCRs may function is that they contain genes encoding lncRNAs that actually activate or repress the transcription of neighbouring families of protein-coding genes. Future studies will be required to determine if other LCRs also transcribe lineage-specific or developmentally regulated lncRNAs and if these lncRNAs activate and/or silence transcription of adjacent families of protein-coding genes. Cultures Human PBMC were isolated from healthy volunteers and stimulated with soluble mouse anti-human CD28 (1 μg ml −1 ; 555725; BD Biosciences) and plate-bound anti-CD3 (10 μg ml −1 ; OKT3 clone American Type Culture Collection), 1 × 10 6 cells ml −1 , under TH1: IL-12 (10 ng ml −1 ), TH2: IL-4 (10 ng ml −1 ) or TH17: IL-1β (20 ng ml −1 ), IL-6 (50 ng ml −1 ), IL-23 (20 ng ml −1 ), IL-21 (100 ng ml −1 ), TGF-β1 (5 ng ml −1 ) and mouse anti-human IFN-γ (10 μg ml −1 ; 554698; BD Biosciences), polarizing conditions. TH1 and TH2 cultures were harvested after 5 days to obtain RNA from primary cultures. TH17 cultures were harvested after 7 days to obtain RNA from primary cultures. After 5 days (TH1 and TH2) or 7 days (TH17), the cultures were restimulated with plate-bound anti-CD3 and harvested 2 days later to obtain RNA from effector cultures. The study was approved by the institutional review board at the Vanderbilt University. Written informed consent was obtained at the time of blood sample collection. RNA isolation and quantitative reverse transcription PCR Total RNA was isolated with Tri-reagent (MRC) and purified with the RNeasy MinElute Cleanup kit (Qiagen) using an on-column DNAse treatment to ensure the absence of genomic DNA contamination according to the manufacturer’s supplied protocol. cDNA was synthesized from the total RNA using the SuperScript III First-Strand Synthesis Kit (Life Technologies) using oligo-dT primers and purified using the Qiagen QiaQuick PCR purification kit. Transcript levels were measured in duplicate by quantitative reverse transcription PCR using TaqMan assays (ABI 7300; Life Technologies) or using SYBR green (Bio-Rad iCycleriQ Real-Time PCR System). Expression levels were calculated relative to GAPDH using the ΔΔCT method. Nuclear and cytoplasmic fractions were isolated from TH2 cultures as described previously [48] . Primer pairs used in SYBR green reactions are listed in Supplementary Table 2 . RNA-seq sample preparation and data analysis RNA was isolated from cultures using Tri-reagent. Library preparation was performed using the Illumina Tru-Seq Stranded mRNA kit. Whole-genome RNA sequencing (RNA-seq) was performed by the Vanderbilt Technologies for Advanced Genomics (VANTAGE) core. 100 bp paired-end reads were generated with an Illumina HiSeq 2500. A quality control was performed at all the stages of sequencing analysis including raw data, alignment and expression quantification [49] using tools such as QC3 (ref. 50 ) and MultiRankSeq [51] . The RNA data were aligned with TopHat2 and gene expression levels were quantified using Cufflinks [38] , [52] . FPKM (reads per kilobase per million reads)-based approaches (Cuffdiff) were used to detect differentially expressed genes [53] . False discovery rate (<0.05) was used to correct for multiple testing. The UCSC genome browser (GRCh37/hg19 build) was used to determine chromosome locations and for other purposes as described in the text. De novo transcriptome assembly was performed on whole-genome RNA-sequencing data from Illumina Tru-Seq Stranded Total RNA libraries using TopHat 2 and Cufflinks using upper quartile normalization (−N) and fragment bias correction (−b). Novel transcripts were assembled from reads prealigned to hg19 using TopHat. Identification of novel lincRNA transcripts was accomplished using established methodologies [43] , [54] . The summarized pipeline for discovery of novel lincRNAs and prediction of transcripts with protein-coding potential is summarized in ( Supplementary Fig. 10 ) [55] , [56] . Cell transfections Human PBMC were incubated for a total of 72 h with 10μg ml −1 plate-bound anti-CD3 (OKT3 clone; American Type Culture Collection), 1 μg ml −1 mouse anti-human CD28 (555725; BD Biosciences) and 10 ng ml −1 IL-4. Cells were transfected after 24 h with Lipofectamine RNAiMax (Life Technologies) using the BLOCK-iT Alexa Fluor Red Fluorescent control siRNA and either an inventoried Silencer Select negative control siRNA or custom designed Silencer Select siRNA for TH2-LCR lncRNA (AC004041.2) according to the supplied protocol. These Silencer Select siRNAs contain a locked nucleic acid chemical modification. After 72 h in culture, the cells were treated with BD GolgiStop protein transport inhibitor and stimulated with 50 nM phorbol 12-myristate 13-acetate and 1 μM ionomycin for an additional 6 h. The cells were fixed, permeabilized and labelled using BD Cytofix and BD PermWash with the following intracellular cytokine markers: APC rat anti-mouse/anti-human IL-5 (1:200 dilution; 554396; BD Biosciences), APC rat anti-human IL-13 (1:200 dilution; 561162; BD Biosciences) or APC rat anti-human IL-4 (1:200 dilution; 554486; BD Biosciences), and the cell surface marker: Pacific Blue mouse anti-human CD4 (1:100 dilution; 558116; BD Biosciences). Flow cytometry experiments were performed on a 5-laser BD LSR Fortessa Special Order Research Product using FACSDiva Software. Supplementary analysis of flow data was performed using FlowJo software (Treestar). RNA-immunoprecipitation RNA-immunoprecipitation (RIP) analysis was performed as described previously [4] , [57] . In brief, TH1 and TH2 primary cultures were harvested, nuclei isolated, lysed and chromatin sheared, followed by incubation with an isotype IgG control antibody (10 μg; sc-2025 (mouse) and sc-2027 (rabbit); Santa Cruz Biotechnology), polyclonal rabbit anti-pan hnRNP (10 μg; sc-30148; Santa Cruz Biotechnology) or monoclonal mouse anti-WDR5 (10 μg; ab56919; Abcam) overnight at 4 °C. Protein A/G beads were added to the lysate and incubated at 4 °C for an additional 3 h. Beads were pelleted, supernatants harvested and beads washed and suspended in Tri-Reagent. RNA bound to the immunoprecipitate was purified following the manufacturer’s supplied protocol (Molecular Research Center). Western blotting analysis for the immunoprecipitation controls was conducted using whole-cell lysates resolved by SDS-polyacrylamide gel electrophoresis and transferred to polyvinylidene difluoride membranes. The membranes were blocked with Odyssey Blocking Buffer (Li-Cor) for 1 h at room temperature and incubated with primary antibodies (polyclonal rabbit anti-pan hnRNP, sc-30148, 1:500 dilution; monoclonal mouse anti-WDR5, ab56919, 2 μg ml −1 dilution) overnight at 4 °C. Membranes were washed and incubated with fluorescence-labelled donkey anti-rabbit IRDye 680 (1:10,000 dilution; 926–3223; Li-Cor) or goat anti-mouse IRDye 800CW (1:10,000 dilution; 926–32210; Li-Cor) antibodies diluted in Odyssey blocking buffer following the manufacturer’s supplied protocol. After secondary incubation, blots were washed and suspended in Tris-buffered saline in a light-protective container immediately before scanning using an Odyssey Infrared Imaging System (Li-Cor) [58] . Chromatin immunoprecipitation ChIP procedures were followed as described using an anti-H3K4-Me3 antibody (10 μg; ab6000; Abcam), anti-WDR5 (10 μg; ab56919; Abcam) and anti-rabbit IgG (10 μg; I5006; Sigma) or anti-mouse IgG (10 μg; sc-2025; Santa Cruz Biotechnology) [33] . Primers used to amplify DNA are listed in Supplementary Table 2 . Quantitative real-time PCR with SYBR green was used to measure DNA after ChIP and DNA purification. Melt curves after amplification showed that primer pairs generated single products. Quantitative ChIP assays were performed in triplicate and results from two or three independent experiments were averaged. Samples with a difference <2.0 in mean Ct value for specific and nonspecific (isotype Ig control) immunoprecipitations were considered nonspecific. Standard curves from the input DNAs were also generated using the different primer pairs. Slopes of these curves were essentially identical. Therefore, we elected not to include input DNA results in our calculations since this only served to add an additional source of error. Relative enrichment was determined using the following formula: 2 (Ct (Ig control)-Ct (antibody-specific IP)) , where Ct (Ig control) was the Ct obtained from the IgG isotype control ChIP and Ct (antibody-specific IP) was the Ct obtained from the antibody-specific ChIP. For example, a mean Ct value of 31 for the isotype control ChIPs and a mean Ct value of 26 for the antibody-specific ChIPs yielded a relative enrichment of 2 (ref. 5 ) or 32. Statistical analysis Unless otherwise indicated, data are expressed as the mean±s.d. of three or more independent experiments. Unless otherwise noted, significance was determined by Student’s t -test using GraphPad Prism Software (La Jolla, CA). P values<0.05 were considered significant. Accession codes. Gene Expression Omnibus GSE 66261 . How to cite this article: Spurlock, C. F. et al . Expression and functions of long noncoding RNAs during human T helper cell differentiation. Nat. Commun. 6:6932 doi: 10.1038/ncomms7932 (2015).